Tectorial membrane travelling waves underlie abnormal hearing inTectbmutant mice Remarkable sensitivity and exquisite frequency selectivity are hallmarks of mammalian hearing, but their underlying mechanisms remain unclear. Cochlear insults and hearing disorders that decrease sensitivity also tend to broaden tuning, suggesting that these properties are linked. However, a recently developed mouse model of genetically altered hearing ( Tectb −/− ) shows decreased sensitivity and sharper frequency selectivity. In this paper, we show that the Tectb mutation reduces the spatial extent and propagation velocity of tectorial membrane (TM) travelling waves and that these changes in wave propagation are likely to account for all of the hearing abnormalities associated with the mutation. By reducing the spatial extent of TM waves, the Tectb mutation decreases the spread of excitation and thereby increases frequency selectivity. Furthermore, the change in TM wave velocity reduces the number of hair cells that effectively couple energy to the basilar membrane, which reduces sensitivity. These results highlight the importance of TM waves in hearing. Our ability to detect and analyse sounds is fundamental to our natural ability to communicate with each other and to navigate through acoustically rich environments. A variety of mechanisms have been demonstrated whereby 'cochlear amplification' [1] , [2] , [3] , [4] , [5] , [6] , [7] , [8] can effectively reduce viscous loss of energy (damping) and thereby increase both sensitivity and frequency selectivity, suggesting that sensitivity and frequency resolution are inextricably linked [1] , [2] , [3] . However, the direct coupling of these remarkable properties is challenged by a recent study of a mouse model of genetically altered hearing ( Tectb −/− ) with decreased sensitivity and strikingly sharpened frequency selectivity [9] , [10] , [11] . Tectb encodes β-tectorin, a glycoprotein that is localized to the tectorial membrane (TM) (ref. 12 ) and the absence of which leads to disruption of the TM's core structure and to significant changes in cochlear function [9] . Targeted deletion of β-tectorin in Tectb −/− mice reduces sensitivity by ∼ 10 dB SPL while simultaneously increasing the sharpness of tuning by about a factor of 2 – 3 at mid to high frequencies; at low frequencies, sensitivity is markedly reduced ( ∼ 50 dB SPL) (ref. 9 ). These physiological changes cannot be explained by a change in effective damping or by any other mechanism that links sharpened frequency selectivity to increased sensitivity. Here, we show that differences in the wave properties of TMs of Tectb −/− and wild-type mice can account for all of the unexplained hearing properties of Tectb −/− mice. According to this mechanism, TM waves coordinate the activities of multiple outer hair cells (OHCs) and thereby have an important role in determining both sensitivity and frequency selectivity of cochlear amplification. At mid and high frequencies, the Tectb mutation reduces the spatial extent and velocity of TM waves, which can reduce cochlear sensitivity while simultaneously sharpening frequency selectivity. At low frequencies, the even greater reduction in TM wave velocity produces an even greater loss of sensitivity. These findings demonstrate mechanisms by which TM waves moderate a balance between sensitivity and exquisite frequency selectivity in mammalian hearing. TM travelling waves in Tectb −/− and wild-type mice To determine how the loss of β-tectorin affects TM waves, we investigated longitudinally propagating waves of radial motion along Tectb −/− and wild-type TMs (see Methods section). TM segments were isolated from the cochleae and suspended between two supports in a fluid-filled wave chamber ( Fig. 1a ). Sinusoidal forces applied in the radial direction at one support generated waves that propagated longitudinally along the TM [13] . These waves were of nanometre scale in amplitude and observed over a broad range of frequencies (1–18 kHz). An optical imaging system using stroboscopic illumination tracked displacement amplitude and phase at multiple points on the surface of the TM. Complex exponentials were fit to the waveforms over 16 phase cycles. These fits contain two free parameters: wavelength ( λ ; distance the wave travels while going through a full cycle of motion) and wave decay constant ( σ ; distance the wave travels before dissipating by a factor of e in amplitude) ( Fig. 1b ). 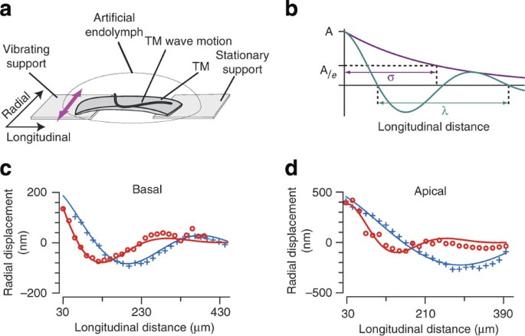Figure 1: Longitudinally propagating waves of radial motion along the TM. (a) TM segments were suspended between two supports separated by 390–480 μm in a wave chamber. Double-headed arrow indicates sinusoidal displacement of vibrating support at audio frequencies. Schematic waveform (green line overlaid on TM) is a displacement snapshot illustrating the wave-like nature of TM motion. (b) Schematic drawing of a decaying wave showing the peak amplitude (A), wave envelope (purple), wave decay constantσand wavelengthλ. (c,d) TM radial displacement versus longitudinal distance across basal and apical TM segments. Radial displacement was measured relative to a point on the TM,∼30 μm from the edge of vibrating support. (c) Wave motion in response to 18-kHz stimulation for basalTectb−/−(red open circles) and wild-type (blue pluses) TMs. Best fitting wave parameter estimates wereσ=110 μm andλ=330 μm forTectb−/−mice, andσ=200 μm andλ=415 μm for wild-type mice. (d) Wave motion in response to 3.5-kHz stimulation for apicalTectb−/−(red open circles) and wild-type (blue pluses) TMs. Best fitting wave parameter estimates wereσ=90 μm andλ=220 μm forTectb−/−mice, andσ=340 μm andλ=560 μm for wild-type mice. Figure 1: Longitudinally propagating waves of radial motion along the TM. ( a ) TM segments were suspended between two supports separated by 390–480 μm in a wave chamber. Double-headed arrow indicates sinusoidal displacement of vibrating support at audio frequencies. Schematic waveform (green line overlaid on TM) is a displacement snapshot illustrating the wave-like nature of TM motion. ( b ) Schematic drawing of a decaying wave showing the peak amplitude (A), wave envelope (purple), wave decay constant σ and wavelength λ . ( c , d ) TM radial displacement versus longitudinal distance across basal and apical TM segments. Radial displacement was measured relative to a point on the TM, ∼ 30 μm from the edge of vibrating support. ( c ) Wave motion in response to 18-kHz stimulation for basal Tectb −/− (red open circles) and wild-type (blue pluses) TMs. Best fitting wave parameter estimates were σ =110 μm and λ =330 μm for Tectb −/− mice, and σ =200 μm and λ =415 μm for wild-type mice. ( d ) Wave motion in response to 3.5-kHz stimulation for apical Tectb −/− (red open circles) and wild-type (blue pluses) TMs. Best fitting wave parameter estimates were σ =90 μm and λ =220 μm for Tectb −/− mice, and σ =340 μm and λ =560 μm for wild-type mice. Full size image Decay constants and wavelengths are reduced in Tectb −/− TMs We captured snapshots of radial motion along TM segments at one phase of a periodic driving signal ( Fig. 1c,d ). At 18 kHz, the waveform of Tectb −/− TM segments excised from the middle to the basal third of the cochlea (referred to as 'basal Tectb −/− TM') had shorter wave decay constants (reduced by ∼ 55%) and wavelengths (reduced by ∼ 20%) than did basal wild-type TMs ( Fig. 1c ). Across the apical segments, Tectb −/− TMs had considerably shorter wave decay constants (reduced by ∼ 75%) and wavelengths (reduced by ∼ 60%) compared with apical wild-type TMs, particularly at low frequencies ( Fig. 1d ). Wave decay constant ( σ ) data were pooled across multiple basal and apical TM segments, further highlighting significant differences between Tectb −/− and wild-type TM samples ( Fig. 2a,b ). Across basal segments, Tectb −/− TMs (11 measurements) had a range of σ -values between 65 and 180 μm at high frequencies (>10 kHz), whereas the range of σ -values for wild-type TMs (16 measurements) were all ≥185 μm ( Fig. 2a ). Across apical segments, the σ -values for Tectb −/− TMs (19 measurements; 45–220 μm) were significantly lower than those for wild-type TMs (15 measurements; ≥190 μm) at frequencies ≥2 kHz ( Fig. 2b ). 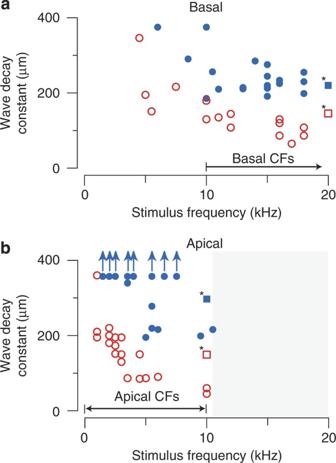Figure 2: Spatial extent of basal and apical TM waves. (a,b) Wave decay constant versus stimulus frequency for basal and apical TMs. Spatial bandwidths of tuning at the 10- and 20-kHz best places calculated from neural tuning curves inTectb−/−(red square with asterisk) and wild-type (blue square with asterisk) mice9are also included. (a) BasalTectb−/−TM segments (n=4 TM preparations; red open circles) had wave decay constant (σ) values between 65 and 180 μm for stimuli >10 kHz. In contrast, theσ-values of basal wild-type TM segments (n=4 TM preparations; blue closed circles) were all ≥185 μm over the same stimulus frequencies (P-value <3.85 × 10−8). Black arrow indicates that characteristic frequencies (CFs) of basal TM segments extend beyond 10 kHz. (b) ApicalTectb−/−TM segments (n=3 TM preparations; red open circles) hadσ-values between 45 and 220 μm for stimuli ≥2 kHz. The wave decay constants of apical wild-type TM segments (n=4 TM preparations; blue closed circles) were typically larger, ranging between 195 and 350 μm, and >350 μm for stimuli ≤7.5 kHz (P-value <1.83 × 10−6). Upward blue arrows indicate thatσ-values were considerably larger than the length of TM in the wave chamber. Double-sided black arrows denote range of CFs corresponding to apical TM segments. The grey shaded region denotes the range of frequencies (>10.5 kHz) when TM motion was significantly attenuated (in the noise floor). Figure 2: Spatial extent of basal and apical TM waves. ( a , b ) Wave decay constant versus stimulus frequency for basal and apical TMs. Spatial bandwidths of tuning at the 10- and 20-kHz best places calculated from neural tuning curves in Tectb −/− (red square with asterisk) and wild-type (blue square with asterisk) mice [9] are also included. ( a ) Basal Tectb −/− TM segments ( n =4 TM preparations; red open circles) had wave decay constant ( σ ) values between 65 and 180 μm for stimuli >10 kHz. In contrast, the σ -values of basal wild-type TM segments ( n =4 TM preparations; blue closed circles) were all ≥185 μm over the same stimulus frequencies ( P -value <3.85 × 10 −8 ). Black arrow indicates that characteristic frequencies (CFs) of basal TM segments extend beyond 10 kHz. ( b ) Apical Tectb −/− TM segments ( n =3 TM preparations; red open circles) had σ -values between 45 and 220 μm for stimuli ≥2 kHz. The wave decay constants of apical wild-type TM segments ( n =4 TM preparations; blue closed circles) were typically larger, ranging between 195 and 350 μm, and >350 μm for stimuli ≤7.5 kHz ( P -value <1.83 × 10 −6 ). Upward blue arrows indicate that σ -values were considerably larger than the length of TM in the wave chamber. Double-sided black arrows denote range of CFs corresponding to apical TM segments. The grey shaded region denotes the range of frequencies (>10.5 kHz) when TM motion was significantly attenuated (in the noise floor). Full size image The reduction in wave decay constants in Tectb −/− TMs ( Fig. 2a,b ) correlates with previously reported reductions in the bandwidth of frequency tuning curves in Tectb −/− mice [9] . The bandwidth of frequency tuning at one cochlear location can be related to the spatial extent of tuning at one stimulus frequency by applying local scaling symmetry (the idea that frequency tuning curves at nearby characteristic frequencies (CFs) are identical when scaled by f CF ) [14] , [15] and then mapping CFs to best cochlear locations [16] . Using this technique, we calculate a 30–50% reduction in spatial bandwidths at the 10 and 20-kHz best locations in Tectb −/− mice with respect to wild types, which is comparable to the reduction in the extent of TM waves in Tectb −/− mice at 10 and 20 kHz ( Fig. 2a,b ). Wave propagation velocities are reduced in Tectb −/− TMs We computed the velocity of wave propagation ( v s ) over a range of stimulus frequencies as the product of frequency and wavelength (2πδ x /δϕ), where δϕ is the phase accumulation between two sites along the TM ( Fig. 3a,b ) and δ x is the longitudinal distance separating those sites. Propagation velocities were generally smaller in Tectb −/− TMs than in wild-type TMs. Although these differences were smaller in basal segments ( Fig. 4a ) than in apical segments ( Fig. 4b ), the differences were statistically significant in both regions. 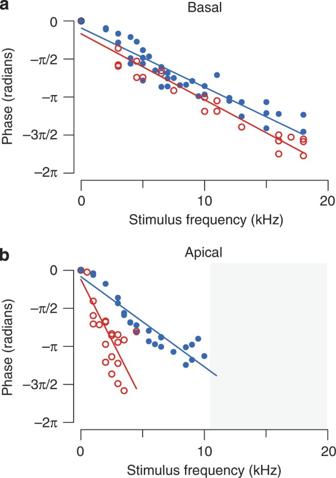Figure 3: Phase vs stimulus frequency for basal and apical TMs. (a) BasalTectb−/−TM segments (n=3 TM preparations; red open circles) accumulated more phase (>10 kHz) than did basal wild-type TMs (n=3 TM preparations; blue closed circles) at a location∼250 μm from the vibrating support. (b) Phase accumulation was greater for apicalTectb−/−TMs (n=4 TM preparations; red open circles) compared with apical wild-type TMs (n=3 TM preparations; blue closed circles) at frequencies above 1 kHz (at∼250 μm location). Lines are linear regression fits to the data. The grey shaded region denotes the range of frequencies (>11 kHz) when TM motion was too small to measure phase differences. Figure 3: Phase vs stimulus frequency for basal and apical TMs. ( a ) Basal Tectb −/− TM segments ( n =3 TM preparations; red open circles) accumulated more phase (>10 kHz) than did basal wild-type TMs ( n =3 TM preparations; blue closed circles) at a location ∼ 250 μm from the vibrating support. ( b ) Phase accumulation was greater for apical Tectb −/− TMs ( n =4 TM preparations; red open circles) compared with apical wild-type TMs ( n =3 TM preparations; blue closed circles) at frequencies above 1 kHz (at ∼ 250 μm location). Lines are linear regression fits to the data. The grey shaded region denotes the range of frequencies (>11 kHz) when TM motion was too small to measure phase differences. 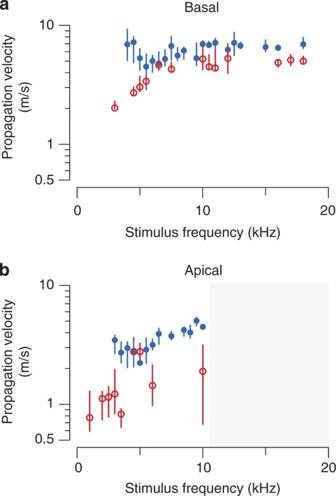Figure 4: Propagation velocity of basal and apical TM waves. Vertical lines mark the interquartile range and circles mark the median wave velocity measured inTectb−/−(red open circles) and wild-type (blue closed circles) TMs at each stimulus frequency (horizontal axis). (a) In basal segments, the median velocities inTectb−/−TMs (n=3 preparations) were smaller than those of wild types (n=7 preparations). Even at high frequencies, when differences were small (10–40%), these differences were statistically significant (P<2×10−4). (b) In apical segments, the median velocities inTectb−/−TMs (n=3 preparations) were significantly smaller (P<0.043) than those of wild types (n=4 preparations), with differences at low frequencies (<5 kHz) of as much as a factor of 6. The grey shaded region denotes the range of frequencies (>11 kHz) when TM motion was too small to measure wave velocity. Full size image Figure 4: Propagation velocity of basal and apical TM waves. Vertical lines mark the interquartile range and circles mark the median wave velocity measured in Tectb −/− (red open circles) and wild-type (blue closed circles) TMs at each stimulus frequency (horizontal axis). ( a ) In basal segments, the median velocities in Tectb −/− TMs ( n =3 preparations) were smaller than those of wild types ( n =7 preparations). Even at high frequencies, when differences were small (10–40%), these differences were statistically significant ( P <2×10 −4 ). ( b ) In apical segments, the median velocities in Tectb −/− TMs ( n =3 preparations) were significantly smaller ( P <0.043) than those of wild types ( n =4 preparations), with differences at low frequencies (<5 kHz) of as much as a factor of 6. The grey shaded region denotes the range of frequencies (>11 kHz) when TM motion was too small to measure wave velocity. Full size image TM material properties account for changes in waves The frequency-dependent wave properties of the TM provide information about the underlying TM material properties. For example, the velocity v s of pure shear waves in an infinite, isotropic, viscoelastic material depends on the shear storage modulus G ' (which characterizes elastic energy stored during parallel motions of the surfaces of a deformable body), the shear viscosity η (which characterizes dissipation of energy) and density ρ , as follows: where ω is the angular frequency of vibration [13] , [17] , [18] . We can use this equation to estimate the material properties of the TM by finding the values of G ′ and η to best fit the measured values of v s (density ρ is taken to be that of water). To account for boundary conditions of the wave chamber and attenuation of wave motion (wave decay constant), we analysed a finite difference model that consists of a longitudinally distributed series of masses coupled to viscous and elastic elements [13] . Sinusoidal stimuli applied to one end of this model of the TM launched travelling waves that were similar to those measured experimentally in wild-type and Tectb −/− TMs. Best fit estimates of the material properties (mean±s.d.) of basal Tectb −/− TMs ( G′ =18±1 kPa, η =0.17±0.06 Pa·s; n =3 TM preparations) were smaller than those of wild-type TMs ( G′ =42±10 kPa, η =0.23±0.07 Pa·s; n =7 TM preparations). For apical TMs, the material properties of Tectb −/− TMs ( G′ =1±0.1 kPa, η =0.12±0.13 Pa·s; n =3 TM preparations) were also reduced with respect to wild-type TMs ( G′ =14±4 kPa, η =0.21±0.12 Pa·s; n =4 TM preparations). Thus, the shear storage modulus G′ was reduced by factors of 2.3 (basal) and 14 (apical) in the TMs of Tectb −/− mutants relative to wild types, whereas viscosity changes were small. We attribute the change in shear storage modulus to disruption of the TM's striated sheet matrix (caused by the absence of β-tectorin), which makes up the core structure of the TM and in which the radial collagen fibres are embedded. Without the striated sheet matrix, the radial collagen fibres lack uniform layout and structural support, thus giving rise to reduced shear storage modulus. In vivo , TM is coupled to hair bundles, attached at the spiral limbus and bound below by a narrow subtectorial fluid space. We tested the effects of these cochlear loads on TM wave propagation in Tectb −/− mice using a finite difference model ( Supplementary Fig. S1a ). We modelled OHC hair bundles as springs, the limbal attachment as an elastic solid and the subtectorial space as a viscous fluid. For physically plausible values of these parameters, the effects of these cochlear loads on wave motion were small ( Supplementary Fig. S1b–d ). Only the limbal attachment had a significant effect on the waves in wild-type and Tectb −/− mice; this effect was to increase the wavelength (by <15%). Results in this study demonstrate that the Tectb mutation alters TM wave properties. These changes in wave properties provide insight into the hearing abnormalities of Tectb −/− mice, which are otherwise difficult to understand. Previously, it was shown that the Tectb mutation leads to sharpened tuning and decreased sensitivity at mid to high frequencies of hearing, and markedly reduced sensitivity at low frequencies [9] . Taken together, these differences in physiological response cannot be explained by a change in effective damping or a simple attenuation in amplification mechanisms. However, this combination of hearing abnormalities is consistent with our measured changes in TM wave velocity and decay constants, as described in the following paragraphs. Because TM waves extend over significant longitudinal distances, these waves would tend to coordinate the activities of many sensory receptors ( ∼ 75 to 150), spanning regions ( ∼ 200 to 400 μm) that correspond to frequencies within an octave of the best frequency [19] . This mechanism could increase the number of OHCs that participate in amplification of narrow-band stimuli and thereby increase cochlear sensitivity by increasing the effective gain of the amplification. The moderate (but statistically significant) decrease in the extent of TM waves in Tectb −/− mice ( Fig. 2a ) could lead to fewer hair cells working in synchrony, thereby causing a moderate decrease in sensitivity ( ∼ 10 dB SPL) at mid to high frequencies [9] , [10] , [11] . Moreover, such a reduction in the coordinated activity of hair cells in Tectb −/− mice would simultaneously lead to an increase in frequency selectivity by reducing the longitudinal spread of excitation, allowing adjacent regions of the cochlea to vibrate at their own local best frequencies. The shorter wave decay constants ( ∼ 55% reduction) in Tectb −/− mice ( Fig. 5 ) would lead to sharpened frequency selectivity, in good agreement with the factor of ∼ 2 increase in sharpness of tuning ( Q 10 dB ) at mid to high frequencies [9] , [10] , [11] . The increased frequency selectivity in the Tectb −/− mutants might be regarded as an improvement in hearing. However, there is a fundamental trade-off between resolution in frequency and resolution in time, and this trade-off implies that increasing frequency selectivity decreases temporal resolution. By this logic, increasing frequency resolution could result in impairment of temporal resolution. The substantial role of longitudinal coupling [20] , [21] , [22] , [23] , [24] , [25] in controlling cochlear tuning and timing is consistent with a recently published cochlear model [18] . 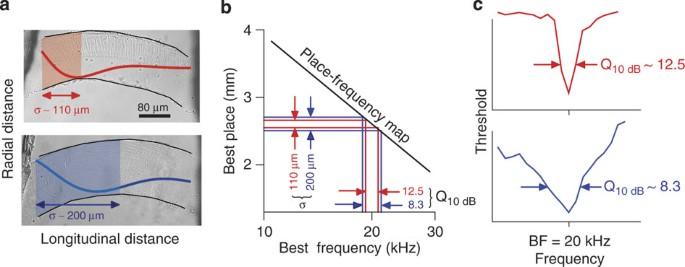Figure 5: Changes in TM wave properties account for abnormal hearing inTectb−/−mice. (a) Light microscope images of typicalTectb−/−(top) and wild-type (bottom) TM samples in the wave chamber. Superimposed waveforms illustrate associated TM wave displacements in response to 18 kHz stimulation (amplitudes exaggerated for clarity). Shaded regions illustrate the decay constantσ, which is the distance over which the wave amplitude decays by a factor ofe(∼110 μm forTectb−/−in red;∼200 μm for wild type in blue). Marginal (top black line) and limbal (bottom black line) boundaries for both TM samples are indicated. (b) Relation between TM decay constants (ordinate) and frequency tuning (abscissa). Distances between pairs of horizontal lines indicate the TM decay constants forTectb−/−(red) and wild-type (blue) TM samples froma. Distances between pairs of vertical lines indicate frequency bandwidths. The relations between spatial and frequency bandwidths are closely approximated by projection onto the sloping line, which indicates the map between best place and best frequency in mouse16. (c) Frequency tuning curves (adapted from Russellet al.9) showing changes in frequency bandwidth in a typicalTectb−/−(red line) and wild-type (blue line) mouse. Arrows indicate bandwidths 10 dB SPL above the most sensitive frequency (20 kHz). Figure 5: Changes in TM wave properties account for abnormal hearing in Tectb −/− mice. ( a ) Light microscope images of typical Tectb −/− (top) and wild-type (bottom) TM samples in the wave chamber. Superimposed waveforms illustrate associated TM wave displacements in response to 18 kHz stimulation (amplitudes exaggerated for clarity). Shaded regions illustrate the decay constant σ , which is the distance over which the wave amplitude decays by a factor of e ( ∼ 110 μm for Tectb −/− in red; ∼ 200 μm for wild type in blue). Marginal (top black line) and limbal (bottom black line) boundaries for both TM samples are indicated. ( b ) Relation between TM decay constants (ordinate) and frequency tuning (abscissa). Distances between pairs of horizontal lines indicate the TM decay constants for Tectb −/− (red) and wild-type (blue) TM samples from a . Distances between pairs of vertical lines indicate frequency bandwidths. The relations between spatial and frequency bandwidths are closely approximated by projection onto the sloping line, which indicates the map between best place and best frequency in mouse [16] . ( c ) Frequency tuning curves (adapted from Russell et al . [9] ) showing changes in frequency bandwidth in a typical Tectb − / − (red line) and wild-type (blue line) mouse. Arrows indicate bandwidths 10 dB SPL above the most sensitive frequency (20 kHz). Full size image Our results show that the absence of β-tectorin also slows the velocity of TM waves ( Fig. 4a,b ). This reduction in velocity could have important implications for cochlear amplification. The concept that cochlear amplification could arise from the interaction of two propagating waves was first described by Hubbard [26] , who showed that wave amplification arises when the velocities of two waves are matched. The small change in TM wave velocity (by a factor of 1.66) that results along basal sections of the cochlea in Tectb −/− mice ( Fig. 4a ) could thereby contribute to the small loss of sensitivity ( ∼ 10 dB SPL) at mid to high frequencies that has been reported for these mice [9] . More importantly, the large change in apical TM wave velocity (by up to a factor of ∼ 6.25; Fig. 4b ) could cause a substantial decrease in sensitivity ( ∼ 50 dB SPL), virtually eliminating amplification at low frequencies. In summary, TM waves constitute a new mechanism that is complementary to those in conventional theories, in which increased gain tends to sharpen tuning [20] . Such a complementary mechanism may be essential for attaining high sensitivity without suffering poor temporal resolution that would result if frequency selectivity were increased excessively. By facilitating high gain with reduced frequency selectivity, TM waves provide a mechanism that functions to balance the relative advantages of sensitivity, frequency selectivity and temporal resolution—all of which are hallmarks of mammalian hearing. Isolated TM preparation TM segments were excised from the cochleae of adult (15–30 g, 4–8 weeks old) Tectb −/− (strain 129SvEv/C57BL6J) and wild-type mice (strains 129SvEv/C57BL6J, B6129F1 and CD-1). No strain-dependent differences were found. Segments (typically 0.5–1 mm in longitudinal length) were isolated from the organ with a sterilized eyelash probe and placed in a fresh artificial endolymph bath (containing 174 mM KCl, 5 mM HEPES, 3 mM dextrose, 2 mM NaCl and 0.02 mM CaCl 2 ) in preparation for wave motion measurements [13] , [27] . TM segments from the low-frequency regions were classified as 'apical' (0–30% from the apex) and those from mid to high frequency regions of the cochlea were classified as 'basal' (40–80% from the apex) [16] , [28] . The care and use of animals in this study were approved by the Massachusetts Institute of Technology Committee on Animal Care. Wave motion measurements Isolated segments of Tectb −/− and wild-type TMs were suspended [13] between the supports of a wave chamber ( Fig. 1a ). One support was attached with epoxy to a piezo-electric actuator (Thorlabs) and loosely coupled to the underlying glass slide. Motion of this vibrating support was examined to ensure uniform sinusoidal motion before each experiment. The second stationary support was firmly fixed to the glass slide with epoxy. To position TM samples in this experiment chamber, the surfaces of the supports were coated with ∼ 0.3 μl of tissue adhesive (Cell Tak; Collaborative Research). Artificial endolymph solution was then perfused in the region of the supports and over the adhesive. The TM segment was then injected into this medium with a small glass-tipped pipette. We used a sterilized eyelash probe to gently manoeuvre the TM into position between the supports. The TM was positioned so that its radial fibres were parallel to the motion of the vibrating support. The suspended region of the TM was approximately 200–300 μm above the surface of the underlying glass slide. The entire suspended TM structure was imaged with a transmitted-light microscope [13] . Optical imaging system The optical system consisted of ×20 and ×40 water immersion objectives (Zeiss Axioplan) with a 0.5 numerical aperture and a transmitted-light condenser (0.8 numerical aperture). Images were collected with a 12 bit, 1024×1024 pixel CCD camera (CAD7-1024A, Dalsa) by strobing the light-emitting diode. The TM segment was illuminated at 16 evenly spaced stimulus phases over several stimulus cycles. The collected images were analysed to determine the first eight harmonics of the periodic motion. We computed the magnitude and phase of radial displacement from the spatial and temporal brightness gradients in the images [29] , [30] . How to cite this article: Ghaffari, R. et al . Tectorial membrane travelling waves underlie abnormal hearing in Tectb mutant mice. Nat. Commun. 1:96 doi: 10.1038/ncomms1094 (2010).